Development and host cell modifications ofPlasmodium falciparumblood stages in four dimensions Blood stages of Plasmodium falciparum cause the pathology of malaria; however, the progression of the parasite through this complex part of the life cycle has never been visualized. In this study, we use four-dimensional imaging to show for the first time the development of individual parasites in erythrocytes and the concomitant host cell modifications. Our data visualize an unexpectedly dynamic parasite, provide a reference for this life cycle stage and challenge the model that protein export in P. falciparum is linked to the biogenesis of host cell modifications termed Maurer's clefts. Our results provide a novel view of the blood-stage development, Maurer's cleft development and protein export in malaria parasites, and open the door to study dynamic processes, drug effects and the phenotype of mutants. Plasmodium falciparum , the causative agent of the most severe form of malaria, infects more than 300 million people annually, of whom more than 2 million die as a result of the disease [1] . Of the multifaceted life cycle in mosquitoes and humans, the continuous asexual development of the parasite in human erythrocytes is solely responsible for the symptoms of malaria. Within the erythrocyte, the parasite develops in its own compartment formed by the parasitophorous vacuolar membrane (PVM). To thrive in this niche, the parasite extensively modifies the host cell through the export of a large number of proteins [2] . The ∼ 48 h asexual development in erythrocytes is complex, with three successive morphological stages [3] . The first phase is termed the 'ring stage'. Ultrastructural work indicates that ring stages are of a biconcave disc or cup shape [4] , [5] . Expression of parasite proteins exported into the host cell peaks in rings [6] , suggesting that host cell modifications are a major task of this stage. The second phase, the 'trophozoite stage', is characterized by rapid parasite growth and the appearance of haemozoin (remnant of digested haemoglobin) in the food vacuole (FV). The mode of haemoglobin internalization is still debated and might include several distinct processes [7] , [8] , [9] . Finally, the parasite enters the 'schizont stage' during which it generates up to 32 daughter merozoites that, after rupture of the host cell, invade new erythrocytes. Only ring stages are apparent in the blood of patients infected with P. falciparum . Trophozoites and schizonts sequester in capillaries of different organs including the brain, a leading cause of malaria-induced morbidity and mortality [10] . Sequestration, and therefore also parasite virulence, depends on the expression of parasite proteins on the host cell surface [11] , [12] , [13] . Parasite-induced vesicular structures in the host cell termed 'Maurer's clefts' are believed to serve as platforms for the trafficking of P. falciparum proteins to the host cell surface [14] . Maurer's clefts can be detected from the late ring stage onwards [5] , [15] and are thought to originate through budding from the PVM or from extensions of the PVM termed the tubovesicular network, their number increasing as the parasite progresses through the cycle [2] , [16] , [17] , [18] , [19] , [20] . This forms the basis for one model that could solve a mechanistic problem in protein export in malaria parasites: although soluble proteins can pass through the recently described translocon at the PVM [21] , it was proposed that transmembrane proteins are loaded into nascent Maurer's clefts forming at the PVM and are thereby exported with the new cleft [2] , [17] , [18] , [22] , [23] . Thus, according to this model, the export of these proteins depends on the continuous genesis of clefts. Alternative models propose small vesicles [24] or soluble protein aggregates [25] that mediate trafficking from the PVM to Maurer's clefts. Although malaria blood stages were described over a century ago [26] , visualization of the growth of these parasites has not been achieved to date. Malaria blood-stage biology was studied in fixed parasites, in live parasites removed from culture or by very short-term analyses under culture conditions such as two-dimensional (2D) time lapse to investigate parasite invasion [27] , [28] , [29] . This limits the perception of the complex development in erythrocytes and hampers the recognition and study of dynamic processes in these stages. This gap in malaria biology contrasts with the detailed knowledge of the parasite's genome, transcriptome and proteome [30] , [31] , [32] , [33] . 3D microscopy over time (4D imaging) has been instrumental in understanding the cell biology in diverse systems [34] , [35] , [36] . Here, we use 4D imaging to show for the first time, to our knowledge, the development and host cell modifications of individual P. falciparum parasites across the erythrocytic cycle. Our data reveal an unexpectedly dynamic parasite and provide indicators for the build-up and completion of host cell modifications, onset of feeding and active preparation for egress. Analysing Maurer's clefts in detail, we unexpectedly find no indication of cleft formation from the PVM but rather that the total number of Maurer's clefts is present shortly after invasion of a new host cell. In accordance, we show that export of different membrane proteins does not require the generation of new clefts but that they are trafficked to readily formed clefts. Our data provide a novel view of the development, host cell modifications and protein export in this important parasite. Establishing time lapse across the P. falciparum blood cycle To visualize the progress of individual parasites through the asexual blood cycle, we used confocal microscopy to collect z -stacks of growing P. falciparum parasites at regular intervals (between 5 and 60 min) over 16–80 h. To establish a framework, we initially followed up wild-type (strain 3D7) parasites at 1-h intervals from invasion to re-invasion using differential interference contrast (DIC) at low resolution. The average time to complete the full cycle was 52.7 h ( n =13; s.d.±2.0 h). A single focus of haemozoin appeared 24 h post invasion (s.d.±1.5 h), suggesting the initiation of the trophozoite stage after roughly half of the cycle. We also observed a distinguishable transition phase from ring to trophozoite ( ∼ 2–4 h), whereas the progress of trophozoites into schizonts was seamless (see below for details). P. falciparum ring stages are mobile and dynamic in shape To obtain a detailed view of blood-stage development, we examined individual parasites in DIC at high resolution by first focusing on their progress through the ring stage. Surprisingly, individual ring stages not only appeared as circular discs but frequently adopted amoeboid forms ( Fig. 1a,b ; Supplementary Movies 1 and 2 , only a single z -section is shown per time point). At other time points, rings appeared as slender forms (arrow Fig. 1a ) that represent laterally positioned disc-shaped parasites ( Supplementary Fig. S1 ). Amoeboid ring stages were previously seen in blood from patients [26] and were predicted on the basis of the morphology of fixed parasites; however, the need for live cell imaging to assess whether this is a regular part of parasite development was noted [15] . Monitoring a large number of cells showed that all rings repeatedly changed between amoeboid and disc-shaped forms ( Fig. 1a,b ; Supplementary Movies 1 and 2 ) and progressed to trophozoites normally ( Supplementary Movie 2 ). Remarkably, ring stages also changed their position within the host cell ( Fig. 1a,b ; Supplementary Movies 1 and 2 ). 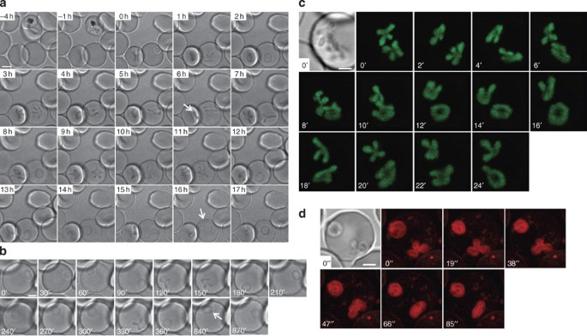Figure 1: Visualization of growing ring-stage parasites. (a) DIC time-lapse imaging (1 h interval) of the development of two ring-stage parasites derived from a single schizont (visible in the first 2 panels). In addition to the ring shape, parasites show amoeboid morphologies. Arrow time point 6 h, laterally seen ring stage; arrow time point 16 h, haemozoin foci. (b) A ring-stage parasite imaged every 30 min showing a higher frequency of regular ring forms. Arrow, haemozoin foci. (a,b) Only a single DIC section of thez-stack acquired at each time point is shown. (c,d) Time-lapse imaging showing the conversion between circular and amoeboid ring forms. Maximum intensity projections of 3D reconstructions of each time point, except for the first panels that show a selected single DIC section for orientation. (c) Cytosolic GFP in REX2ΔTM-GFP-expressing parasites, 2 min interval. (d) Bodipy-TR-C5-ceramide-stained 3D7 parasites, 19 s interval. Scale bars, 3 μm (a) and 2 μm (b–d). Figure 1: Visualization of growing ring-stage parasites. ( a ) DIC time-lapse imaging (1 h interval) of the development of two ring-stage parasites derived from a single schizont (visible in the first 2 panels). In addition to the ring shape, parasites show amoeboid morphologies. Arrow time point 6 h, laterally seen ring stage; arrow time point 16 h, haemozoin foci. ( b ) A ring-stage parasite imaged every 30 min showing a higher frequency of regular ring forms. Arrow, haemozoin foci. ( a , b ) Only a single DIC section of the z -stack acquired at each time point is shown. ( c , d ) Time-lapse imaging showing the conversion between circular and amoeboid ring forms. Maximum intensity projections of 3D reconstructions of each time point, except for the first panels that show a selected single DIC section for orientation. ( c ) Cytosolic GFP in REX2ΔTM-GFP-expressing parasites, 2 min interval. ( d ) Bodipy-TR-C 5 -ceramide-stained 3D7 parasites, 19 s interval. Scale bars, 3 μm ( a ) and 2 μm ( b–d ). Full size image To observe the conversion between round and irregular forms, we used parasites expressing cytosolic green fluorescent protein (GFP) (REX2ΔTM-GFP [37] , a cell line showing indistinguishable fluorescence to parasites expressing GFP alone [38] but which was used because of superior fluorescence) to generate successive 3D reconstructions of growing ring stages with short time intervals. Within tens of seconds to minutes, ring stages gradually changed between forms through protrusion and retraction of lobes from the main ring body ( Fig. 1c ). 3D rotations illustrate the successive amoeboid ( Supplementary Movie 3 , time point 0) and biconcave disc shape ( Supplementary Movie 4 , time point 12 min) of the parasites shown in Figure 1c . Similar results were obtained in wild-type parasites stained with the membrane marker Bodipy-TR-C 5 -ceramide ( Fig. 1d ). A rare parasite remaining stationary within its host cell showed consecutive protrusions in similar positions ( Supplementary Movie 5 ), but because of the mobility of rings it was not possible to establish whether this can be generalized. Taken together, these results suggest the capacity for active cell shape change of intracellular blood stages and show that ring stages move freely in the host cell. Although filamentous actin and several regulators of actin polymerization that mediate cell shape changes [39] have remained elusive in malaria blood stages [40] , the morphology changes of ring stages resembling filopodia-like extensions are an indication of a functional and regulated cytoskeleton. To test a possible role of actin in these shape changes, we counted the number of round and amoeboid forms when parasites were grown for 1 h in the presence of the F-actin stabilizer jasplakinolide. Jasplakinolide concentrations previously used in P. falciparum blood stages [41] resulted in a strong reduction in the number of amoeboid forms ( Fig. 2a ). Reducing the concentration 20-fold (0.05 μM) still showed a clear effect, whereas a 40-fold reduction showed levels of amoeboid forms similar to the dimethylsulphoxide control (DMSO) ( Fig. 2b,c ). This indicates a role for actin in these cell shape changes. Surprisingly, the actin filament destabilizer cytochalasin D had no effect ( Fig. 2d ). This may be due to the fact that most of parasite actin is already present in globular form [40] . The tubulin inhibitors taxol and colchicine showed no effect ( Supplementary Fig. S2a,b ); however, the myosin inhibitor 2,3-butanedione monoxime (BDM) showed reversal of parasites into the round state at its lower activity spectrum (5 mM; Supplementary Fig. S2c ). However, as BDM is known to have off-target effects [42] , inhibition of parasite myosin is only one possible interpretation for this result but would be in agreement with a role of myosin together with actin in the observed cell shape changes. 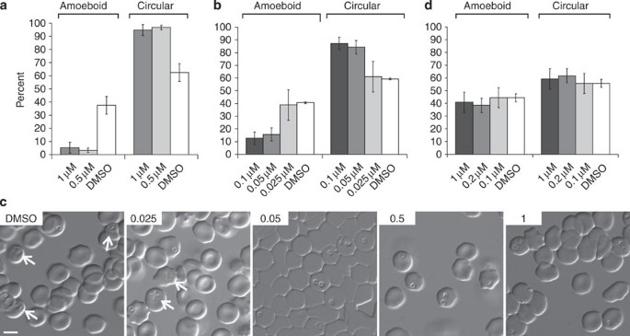Figure 2: Treatment of ring-stage parasites with drugs having an effect on actin. Parasites were grown for 1 h with the indicated concentrations of jasplakinolide and the number of amoeboid and round stages was counted (indicated in percent) using previously used concentrations of jasplakinolide in malaria blood stages41(a) or jasplakinolide in its lower activity range (b). At least 100 cells were counted per concentration and experiment (n=4). Values are shown as mean±s.d. (c) Representative images of jasplakinolide-treated parasites (concentrations indicated in μM). Amoeboid rings are indicated by arrows. Scale bar, 5 μm. (d) Parasites were grown for 1 h with the concentrations of cytochalasin D indicated and analysed as ina. Values are shown as mean±s.d. (n=4). Figure 2: Treatment of ring-stage parasites with drugs having an effect on actin. Parasites were grown for 1 h with the indicated concentrations of jasplakinolide and the number of amoeboid and round stages was counted (indicated in percent) using previously used concentrations of jasplakinolide in malaria blood stages [41] ( a ) or jasplakinolide in its lower activity range ( b ). At least 100 cells were counted per concentration and experiment ( n =4). Values are shown as mean±s.d. ( c ) Representative images of jasplakinolide-treated parasites (concentrations indicated in μM). Amoeboid rings are indicated by arrows. Scale bar, 5 μm. ( d ) Parasites were grown for 1 h with the concentrations of cytochalasin D indicated and analysed as in a . Values are shown as mean±s.d. ( n =4). Full size image The transition from ring to trophozoite A critical step in the life cycle of P. falciparum is the transition from the ring to the cytoadherent trophozoite stage. 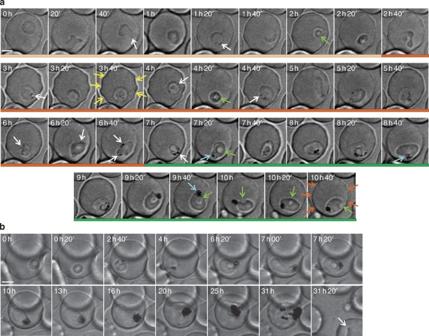Figure 3: The development of the parasite from late ring stage to egress. Only a single DICz-section of the stacks acquired at each time point is shown. (a) 3D7 parasite growing from late ring to the trophozoite stage viewed every 20 min. Live cycle phases are indicated below the panel: sand colour, ring; orange, transition to the trophozoite stage; green, trophozoite. Arrows indicate the following (shown in selected images only): green, cavity; white, multiple haemozoin foci; cyan, single haemozoin focus. The transient echinocytosis of the infected host cell is apparent in a comparison with a time point before and after relief of the echinocytosis as highlighted by arrows during (yellow) and after (orange) echinocytosis. (b) Selected time points of the DIC time-lapse series (20 min interval) shown inSupplementary Movie 6of a parasite growing from late ring to reinvasion. The white arrow shows a ring stage derived from reinvasion after rupture. Scale bar, 2 μm. This phase is shown in Figure 3a and Supplementary Movie 2 , and the complete development of the parasite from the ring stage onwards is shown in Supplementary Movie 6 (selected frames are shown in Fig. 3b ). Towards the end of the ring stage, parasites temporarily condensed into rings of reduced diameter. In DIC, these forms contained a clearly distinguishable circular area in their cytoplasm ( Fig. 3a,b ) that represents a central cavity resulting from a pronounced cup shape of the parasite as opposed to the more spread-out disc shape predominating in earlier stages (compare Supplementary Figs S1 and S3a,b ). Further progressing into the cycle, the condensed late ring stages alternated with more spread-out irregular forms that often contained multiple small foci of haemozoin in their periphery (arrows, Figs 3a and 4a ), suggestive of multiple small FVs and an increased metabolic rate. Figure 3: The development of the parasite from late ring stage to egress. Only a single DIC z -section of the stacks acquired at each time point is shown. ( a ) 3D7 parasite growing from late ring to the trophozoite stage viewed every 20 min. Live cycle phases are indicated below the panel: sand colour, ring; orange, transition to the trophozoite stage; green, trophozoite. Arrows indicate the following (shown in selected images only): green, cavity; white, multiple haemozoin foci; cyan, single haemozoin focus. The transient echinocytosis of the infected host cell is apparent in a comparison with a time point before and after relief of the echinocytosis as highlighted by arrows during (yellow) and after (orange) echinocytosis. ( b ) Selected time points of the DIC time-lapse series (20 min interval) shown in Supplementary Movie 6 of a parasite growing from late ring to reinvasion. The white arrow shows a ring stage derived from reinvasion after rupture. Scale bar, 2 μm. 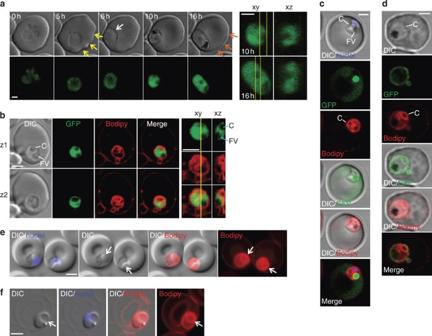Figure 4: The central cavity in malaria parasites. (a) DIC (singlez-section, top row) and maximum intensity projection of cytosolic GFP (green, bottom row) of selected time points of a REX2ΔTM-GFP-expressing parasite growing from late ring to the trophozoite stage. Echinocytosis is highlighted with arrows during (yellow) and after (orange) echinocytosis. An enlargement with axyandxzprojection of the 10 h and 16 h time points show that the circular area visible in the parasite cytoplasm by DIC lacks GFP. The region between the yellow lines was used for the cross-section inxz. (b) Two sections (z1 and z2) through a growing REX2ΔTM-GFP (green)-expressing parasite stained with Bodipy-TR-C5-ceramide (red). The cavity (C) and the food vacuole (FV) are highlighted in the z1 DIC section and in axyandxzprojection of a 3D reconstruction of this infected erythrocyte; the yellow line marks the region used for thexzsection. (c) A parasite of a line exporting GFP into the host cell and stained with Bodipy-TR-C5-ceramide (red) indicates that the cavity contains host cell cytosol. A single confocalz-section is shown. Note that the nucleus (blue) and the FV (filled with reinternalized GFP) are clearly distinct from the cavity. (d) A cell line exporting GFP into the PV shows a fluorescence pattern similar to Bodipy-TR-C5-ceramide staining (red). A single confocal section is shown. (e)P. bergheiparasites stained with Bodipy-TR-C5-ceramide (red) show a cavity (white arrows) similar to the one seen inP. falciparumthat appears as a notch in the parasite in DIC. (f) Tetanolysin lysis ofP. berghei-infected erythrocytes shows that the cavity is part of the parasite body. (c,e,f) Parasite nuclei stained with DAPI are in blue. Scale bars, 1 μm (a), 2 μm (b–f). Full size image Figure 4: The central cavity in malaria parasites. ( a ) DIC (single z -section, top row) and maximum intensity projection of cytosolic GFP (green, bottom row) of selected time points of a REX2ΔTM-GFP-expressing parasite growing from late ring to the trophozoite stage. Echinocytosis is highlighted with arrows during (yellow) and after (orange) echinocytosis. An enlargement with a xy and xz projection of the 10 h and 16 h time points show that the circular area visible in the parasite cytoplasm by DIC lacks GFP. The region between the yellow lines was used for the cross-section in xz . ( b ) Two sections (z1 and z2) through a growing REX2ΔTM-GFP (green)-expressing parasite stained with Bodipy-TR-C 5 -ceramide (red). The cavity (C) and the food vacuole (FV) are highlighted in the z1 DIC section and in a xy and xz projection of a 3D reconstruction of this infected erythrocyte; the yellow line marks the region used for the xz section. ( c ) A parasite of a line exporting GFP into the host cell and stained with Bodipy-TR-C 5 -ceramide (red) indicates that the cavity contains host cell cytosol. A single confocal z -section is shown. Note that the nucleus (blue) and the FV (filled with reinternalized GFP) are clearly distinct from the cavity. ( d ) A cell line exporting GFP into the PV shows a fluorescence pattern similar to Bodipy-TR-C 5 -ceramide staining (red). A single confocal section is shown. ( e ) P. berghei parasites stained with Bodipy-TR-C 5 -ceramide (red) show a cavity (white arrows) similar to the one seen in P. falciparum that appears as a notch in the parasite in DIC. ( f ) Tetanolysin lysis of P. berghei -infected erythrocytes shows that the cavity is part of the parasite body. ( c , e , f ) Parasite nuclei stained with DAPI are in blue. Scale bars, 1 μm ( a ), 2 μm ( b – f ). Full size image An unexpected change accompanying the transition to the trophozoite stage was a usually very mild (in some cases barely perceptible), but in rare cases more pronounced, echinocytosis of the host cell that resolved over the next few hours ( Figs 3a and 4a ). This echinocytosis was much milder than that seen after parasite invasion [28] , [29] , but its occurrence always during the same life cycle stage suggests a physiological process. In the final phase of the transition to the trophozoite stage, the parasite settled into a fixed position in the periphery of the erythrocyte ( Fig. 3a , Supplementary Movie 2 ). At this stage, parasites resembled the condensed forms seen towards the end of the ring stage, but contained haemozoin that over time became concentrated in one larger focus indicative of a single FV ( Fig. 3a ). This agrees with observations indicating multiple digestive compartments in rings, whereas only a single large FV is found in later stages [3] , [7] . No evidence was found for the closure of the central cavity, a process termed the 'big gulp' that was proposed to create the single FV of trophozoites [8] . We find that the central cavity persists into the mid-trophozoite stage as a structure independent of the FV or the multiple FVs in earlier stages ( Figs 3 and 4a , Supplementary Movies 2 and 6 ). A cavity is a prominent feature of malaria blood stages The persistence of the central cavity into later-stage parasites was unexpected and prompted a closer analysis of this structure. Depending on its position, the cavity appeared either as a circular area in the parasite or as a notch breaking the parasite periphery ( Supplementary Fig. S3c–g ). In Bodipy-TR-C 5 -ceramide-stained REX2ΔTM-GFP-expressing parasites it was detectable as a membrane delineated area that lacked cytosolic GFP ( Fig. 4b , Supplementary Fig. S3e ). This was confirmed using the cell line expressing GFP alone [38] ( Supplementary Fig. S3f ). Parasites expressing GFP in the host cell cytosol (using the REX3 export motif [22] , [43] ) showed fluorescence in the cavity ( Fig. 4c ), whereas a cell line expressing GFP in the PV (using the EXP1 signal peptide [44] ) showed staining similar to Bodipy-TR-C 5 -ceramide ( Fig. 4d ), indicating that the cavity represents an invagination of the PVM and the parasite plasma membrane, forming a space filled with host cell cytosol. Interestingly, a similar structure referred to as 'spherical structure' was recently described [7] . We next asked whether the cavity is a general feature of malaria parasites. Analysis of the blood stages of the rodent malaria parasite P. berghei revealed a similar Bodipy-TR-C 5 -ceramide-delineated area that in DIC appeared as a circular gap in the periphery of the parasite ( Fig. 4e ). When P. berghei -infected erythrocytes were lysed with tetanolysin to release the host cell cytosol, the cavity in the parasite body was clearly revealed ( Fig. 4f ). These data suggest that the cavity is a general feature of Plasmodium blood stages and may constitute the translucent area seen in Giemsa-stained trophozoites in diverse malaria species. It is noteworthy to mention that Bodipy-TR-C 5 -ceramide appears enriched in the cavity ( Supplementary Movie 7 ), possibly indicating a distinctive lipid composition. The trophozoite stage Initially, the single FV in young trophozoites changed its position in a whirling motion around the central cavity ( Supplementary Movie 2 ). Over the next hours, the FV settled on one side of the parasite and trophozoites rapidly increased in size. They changed between roundish and elongated forms ( Fig. 3b , Supplementary Movies 2 and 6 ) but differed from the more regular round appearance of living trophozoites viewed at ambient temperature (compare Supplementary Fig. S3c,e ). Growing trophozoites showed indications of cell polarity: the FV remained in the periphery of one of the narrow sides of the parasite with elongations occurring along the longitudinal axis ( Fig. 3b ). The central cavity was still visible but less pronounced in elongated parasites, and showed a preference for the narrow side opposite the FV in more mature trophozoite stages ( Supplementary Movies 2 and 6 ). Late trophozoite to egress During development to the schizont stage, the cavity disappeared and parasites steadily grew in size without profound morphological changes. The FV moved from the periphery to a more central position (generally 10–15 h before rupture), and small vesicle-like structures appeared in the parasite. At 2–3 h before rupture, parasites occupied most of the host cell and showed a more ruffled appearance ( Fig. 3b , Supplementary Movies 1 and 6 ). On rupture, merozoites rapidly dispersed ( Supplementary Movie 1 ). To visualize the formation of merozoites, we used parasites expressing a GFP-tagged protein residing in the parasitophorous vacuole (REX2ΔTM+SP-GFP [37] ). This revealed that merozoite formation is a fast process: the first parasite internal traces of GFP suggestive of invagination of the parasite plasma membrane were visible 3–4 h before rupture, and within 2 h before rupture the parasitophorous vacuole delineated individual merozoites ( Fig. 5a ). 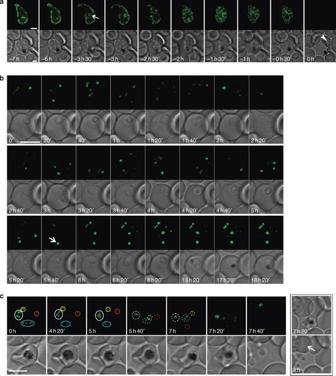Figure 5: Time of merozoite formation and three states of Maurer's clefts. (a) Time-lapse analysis of parasites expressing a GFP-tagged protein in the parasitophorous vacuole (REX2ΔTM+SP-GFP). Top row: selected singlez-section of GFP fluorescence per time point; bottom row: corresponding DIC sections. The GFP image is enlarged in relation to the DIC image. First appearance of parasite internal GFP fluorescence is indicated by a white arrow. The white arrowhead shows a reinvaded parasite after schizont rupture. (b) Time-lapse series (20 min interval) of a REX2-GFPmal7p1.170-expressing parasite. Upper rows: maximum intensity projection of 3D reconstructions of GFP fluorescence labelling Maurer's clefts; bottom rows: single DICz-section of the corresponding time point. The first arrested cleft is indicated with a white arrow (5 h 40′); general arrest of clefts occurred 20 min later. (c) Selected time points of 4D imaging (20 min interval) of a REX2-GFP-expressing schizont. Top and bottom rows are as in (b). The box shows lower magnifications to document reinvasion (white arrow). Different groups of clefts are marked with colour-coded circles to show their changing position. The broken lines encircle clefts that cannot be assigned with certainty. In the last time point before rupture, no assignment could be made. Scale bars, 2 μm (a), 5 μm (b,c). Figure 5: Time of merozoite formation and three states of Maurer's clefts. ( a ) Time-lapse analysis of parasites expressing a GFP-tagged protein in the parasitophorous vacuole (REX2ΔTM+SP-GFP). Top row: selected single z -section of GFP fluorescence per time point; bottom row: corresponding DIC sections. The GFP image is enlarged in relation to the DIC image. First appearance of parasite internal GFP fluorescence is indicated by a white arrow. The white arrowhead shows a reinvaded parasite after schizont rupture. ( b ) Time-lapse series (20 min interval) of a REX2-GFP mal7p1.170 -expressing parasite. Upper rows: maximum intensity projection of 3D reconstructions of GFP fluorescence labelling Maurer's clefts; bottom rows: single DIC z -section of the corresponding time point. The first arrested cleft is indicated with a white arrow (5 h 40′); general arrest of clefts occurred 20 min later. ( c ) Selected time points of 4D imaging (20 min interval) of a REX2-GFP-expressing schizont. Top and bottom rows are as in ( b ). The box shows lower magnifications to document reinvasion (white arrow). Different groups of clefts are marked with colour-coded circles to show their changing position. The broken lines encircle clefts that cannot be assigned with certainty. In the last time point before rupture, no assignment could be made. Scale bars, 2 μm ( a ), 5 μm ( b , c ). Full size image Maurer's clefts show three phases during blood-stage development Next, we analysed parasite host cell modifications focusing on Maurer's clefts using the integral Maurer's cleft protein REX2 fused to GFP [37] (see Supplementary Movie 7 for a 3D representation of Maurer's clefts). REX2-GFP was only detectable from the young trophozoite stage onwards. Unexpectedly, follow-up of these cells through the remainder of the cycle showed that the position and number of Maurer's clefts in individual cells remained constant until shortly before rupture ( Supplementary Fig. S4 ). To obtain a more comprehensive picture of Maurer's cleft development, we exchanged the crt promoter-driving expression of REX2-GFP with that of a previously described ring stage-specific gene (Mal7P1.170) [45] . Unlike REX2-GFP crt , REX2-GFP mal7P1.170 was already detectable in ring stages. Interestingly, in contrast to later stages, Maurer's clefts were highly mobile in rings ( Supplementary Movies 8 and 9 ). With transition to the trophozoite stage, the position of the clefts became fixed and remained unchanged in further development, as seen with REX2-GFP crt ( Fig. 5b ; Supplementary Fig. S5 ). Transition between mobile and immobile clefts occurred in less than an hour and in the same life cycle phase (but not necessarily coinciding) with fixation of the position of the parasite in the host cell. In this time frame, some clefts stopped moving earlier than others, with smaller rearrangements still occurring ( Fig. 5b ; Supplementary Fig. S5 ). The subsequent rapid growth suggests that arrest of parasite and cleft movement signify completion of host cell modifications. In the final stages of the life cycle, a third phase of cleft development was observed. In many cells, the spatial arrangement of clefts collapsed 2–4 h before merozoite egress ( Fig. 5c ). This suggests an active process of disassembling host cell modifications, which coincides with the time of merozoite formation ( Fig. 5a ). Cleft formation is early and not required for protein export The lack of detectable cleft formation from the early trophozoite onwards has important implications for protein export. It suggests that, at least after this stage, exported membrane proteins reach the clefts in other ways than through the formation of new clefts [2] , [17] , [18] , [22] . To confirm this, we used parasites expressing REX2 fused to the irreversibly photoconvertible protein Dendra2 (refs 46 , 47 ). Complete conversion of REX2-Dendra2 at a single cleft from green to red ( Fig. 6a , white box) showed that, with parasite growth, the red cleft accumulated new green fluorescence ( Fig. 6a , arrows). This signifies arrival of unconverted REX2-Dendra2 from the parasite unless the protein was derived from neighbouring clefts. To test this possibility, we converted REX2-Dendra2 in multiple clefts of infected cells and checked whether the converted protein distributed to other clefts. Although intensifying the red signal consistently revealed minimal transfer of red label to other clefts after 10 h ( Fig. 6b ), the accumulation of new green fluorescence over time was much more prominent, indicating that the majority of green label was derived from newly exported protein. Conversion of the majority of the clefts of infected cells confirmed this: although in some of these cells low-level transfer of red fluorescence to unconverted clefts was detectable already after 5 h ( Supplementary Fig. S6a ), this was not the case in other cells, and these cells still showed an increase in the proportion of green label ( Fig. 6c ). Thus, the majority of new protein arriving in converted clefts derives from the parasite; however, some limited lateral transfer between clefts seems to be possible. One explanation for this would be the conversion of green to red by the viewing laser. However, unconverted neighbouring cells in the same imaging area never showed red staining ( Supplementary Fig. S6b ), rendering this possibility unlikely. In conclusion, these data show that membrane-associated proteins can reach readily formed clefts. This would also be supported by laterally transferred protein because there is no lipid continuum between clefts [48] , posing a similar mechanistic problem to PVM to cleft transfer. 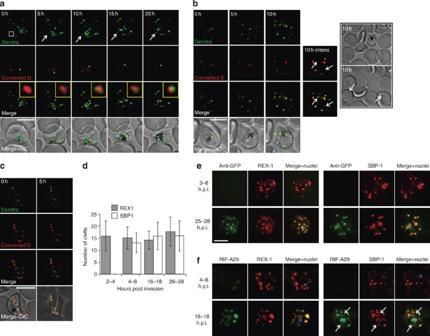Figure 6: Export of membrane proteins is independent of cleft formation. (a) Complete conversion of the fluorescence in a single cleft in a REX2-Dendra2-expressing parasite from green (top panel, white box) to red (second panel). Panels were merged as indicated; the inlay shows an enlargement of the merged red and green fluorescence of the converted cleft. Fluorescence images are maximum intensity projections of 3D reconstructions; DIC is from singlez-sections. The asterisk shows fluorescence derived from FV reflection. (b) Projections of 3D reconstructions of a REX2-Dendra2-expressing parasite where a main part of the four most strongly fluorescing clefts were converted to red. An intensified image of the red fluorescence after 10 h and its merge with the green channel are shown to the right (10 h intens). Arrows indicate red fluorescence in unconverted clefts. This parasite led to two reinvasions in the course of the experiment (right DIC panel). (c) A parasite in which the majority of clefts were converted showed no transfer of red fluorescence. (d) Average number of clefts per cell and time point in a highly synchronous culture as determined by IFA using the cleft markers REX1 and SBP1. SBP1 was not detectable in the first time point. Values are mean±s.d.; one of three representative experiments is shown. (e,f) IFA showing that in REX2-GFPcrt-expressing parasites (e) and 3D7 (f), early clefts contain REX1 and SBP1 but not REX2-GFPcrt(e, upper panels) or RIFIN A29(RIF-A29,f, upper panels). On progress of the culture to the trophozoite stage, the clefts containing REX1 and SBP1 now also contain REX2-GFPcrt(e, lower panel) and RIFIN A29(f, lower panel). Dots positive for RIFIN A29only, found in∼50% of cells, are indicated by white arrows. Scale bars, 5 μm; h.p.i., hours post invasion. Figure 6: Export of membrane proteins is independent of cleft formation. ( a ) Complete conversion of the fluorescence in a single cleft in a REX2-Dendra2-expressing parasite from green (top panel, white box) to red (second panel). Panels were merged as indicated; the inlay shows an enlargement of the merged red and green fluorescence of the converted cleft. Fluorescence images are maximum intensity projections of 3D reconstructions; DIC is from single z -sections. The asterisk shows fluorescence derived from FV reflection. ( b ) Projections of 3D reconstructions of a REX2-Dendra2-expressing parasite where a main part of the four most strongly fluorescing clefts were converted to red. An intensified image of the red fluorescence after 10 h and its merge with the green channel are shown to the right (10 h intens). Arrows indicate red fluorescence in unconverted clefts. This parasite led to two reinvasions in the course of the experiment (right DIC panel). ( c ) A parasite in which the majority of clefts were converted showed no transfer of red fluorescence. ( d ) Average number of clefts per cell and time point in a highly synchronous culture as determined by IFA using the cleft markers REX1 and SBP1. SBP1 was not detectable in the first time point. Values are mean±s.d. ; one of three representative experiments is shown. ( e , f ) IFA showing that in REX2-GFP crt -expressing parasites ( e ) and 3D7 ( f ), early clefts contain REX1 and SBP1 but not REX2-GFP crt ( e , upper panels) or RIFIN A 29 (RIF-A29, f , upper panels). On progress of the culture to the trophozoite stage, the clefts containing REX1 and SBP1 now also contain REX2-GFP crt ( e , lower panel) and RIFIN A 29 ( f , lower panel). Dots positive for RIFIN A 29 only, found in ∼ 50% of cells, are indicated by white arrows. Scale bars, 5 μm; h.p.i., hours post invasion. Full size image These findings do not exclude the possibility that cleft formation occurs in earlier stages and mediates protein export. The rapid movement of clefts in rings precludes time-lapse analysis to test this. We therefore counted the number of clefts per cell at different time points of highly synchronous parasite cultures (1.5–3 h time window) using Maurer's cleft markers REX1 (ref. 49 ) and SBP1 (ref. 50 ). There was no increase in the average number of clefts per cell as the population of parasites grew from early ring to the trophozoite stage ( Fig. 6d ). This suggests that no or few clefts are formed from early ring to the trophozoite stage. These experiments also demonstrated that clefts are already present much earlier than previously thought [5] , [15] , with REX1 appearing 2–4 h after invasion and SBP1 4–6 h post invasion ( Fig. 6d–f ). Importantly, other cleft proteins were not detectable in early-stage parasites but only in later-stage parasites (see below), a fact that can be used to confirm that protein export is independent of cleft formation: if export required the formation of new clefts, these later expressed proteins would be missing from early formed clefts, leading to a mixed population of Maurer's clefts, each cleft displaying the proteins expressed at the time of its formation. In contrast, if export was independent of cleft formation (as suggested by our data), clefts would continuously receive protein, leading to a homogeneous distribution of antigens in all clefts. We tested these two possibilities using endogenous REX1 and SBP1 as early cleft proteins, and REX2-GFP crt (in transgenic parasites) and endogenous RIFIN-A 29 (ref. 51 ; in 3D7 parasites) as later-stage Maurer's cleft proteins. As expected, the clefts in early stages contained only the early markers ( Fig. 6e,f ). In contrast, later stages were positive for all four antigens ( Fig. 6e,f ). Crucially, in later stages all antigens occupied the same clefts ( Fig. 6e,f ), demonstrating that the clefts initially containing REX1 and SBP1 accumulated the other proteins later on. This establishes that export occurred without cleft formation. For RIFIN-A 29 , ∼ 50% of cells contained a low proportion of dots (usually one or two and always in the lower intensity range) positive for RIFIN-A 29 alone ( Fig. 6f , arrows). These signals might therefore represent vesicles to or from Maurer's clefts or a minimal number of newly formed clefts. This study shows the development of P. falciparu m blood stages by long-term time-lapse imaging, providing a reference for the asexual life cycle in erythrocytes ( Fig. 7 ). This includes the finding of a stage of profound changes that represents the major turning point in the cycle that we designated 'transition to the trophozoite', where the highly mobile but slowly growing ring-stage parasite settles into the stationary, haemoglobin-ingesting and fast-growing trophozoite. During this phase, Maurer's clefts change from a mobile to a fixed state, and a very mild echinocytosis of the host cell occurs. Transition to the trophozoite coincides temporally with the appearance of the cytoadherence protein PfEMP1 on the host cell surface [52] , leading to sequestration in vivo [10] . The echinocytosis might therefore indicate processes of surface remodelling that affect the homeostasis of the erythrocyte or changes to the host cell cytoskeleton. The arrest of Maurer's clefts may aid protein export to the host cell surface. This likely reflects a close coordination of host cell modifications with changes in parasite morphology, as survival of the rapidly growing trophozoite depends on sequestration [10] . In a similar concerted manner, we find that segmentation of merozoites coincides with the time Maurer's clefts collapse, indicating active dismantling of host cell modifications to facilitate egress. 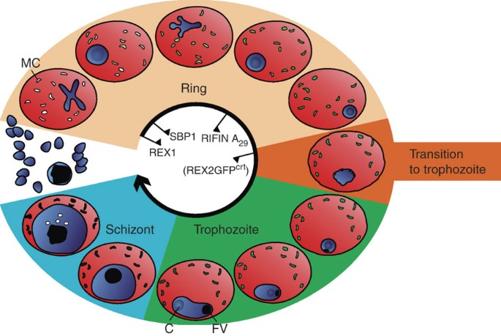Figure 7: Model of the asexual cycle ofP. falciparumin erythrocytes. The ring stage (sand coloured) was defined as the stage at which parasites cycle between disc and amoeboid forms, change position within the cell, do not contain haemozoin and Maurer's clefts are mobile; transition stage to trophozoite (orange) as the time when parasites cycle between condensed and irregular forms with multiple small haemozoin foci and the host cell shows a very mild echinocytosis; the trophozoite stage (green) was defined as the stage after parasites and Maurer's clefts (MC) had settled into a fixed position (indicating completion of host cell modification) and the haemozoin was found in a single FV (FV), after which the amount of haemozoin increased rapidly (suggestive of a high metabolic rate); transition to the schizont (blue) was seamless, with disappearance of the cavity (C), move of the FV to a more central position and appearance of vesicle-like structures (white circles). Time of expression start for the different MC antigens, REX1, SBP1, REX2-GFPcrt(in brackets to denote episomal expression) and RIFIN-A29, is indicated by arrows. The cascade of different proteins arriving at these structures is signified by different shading of MC. Relative timing of stages and appearance of antigens in the MC is approximate. Figure 7: Model of the asexual cycle of P. falciparum in erythrocytes. The ring stage (sand coloured) was defined as the stage at which parasites cycle between disc and amoeboid forms, change position within the cell, do not contain haemozoin and Maurer's clefts are mobile; transition stage to trophozoite (orange) as the time when parasites cycle between condensed and irregular forms with multiple small haemozoin foci and the host cell shows a very mild echinocytosis; the trophozoite stage (green) was defined as the stage after parasites and Maurer's clefts (MC) had settled into a fixed position (indicating completion of host cell modification) and the haemozoin was found in a single FV (FV), after which the amount of haemozoin increased rapidly (suggestive of a high metabolic rate); transition to the schizont (blue) was seamless, with disappearance of the cavity (C), move of the FV to a more central position and appearance of vesicle-like structures (white circles). Time of expression start for the different MC antigens, REX1, SBP1, REX2-GFP crt (in brackets to denote episomal expression) and RIFIN-A 29 , is indicated by arrows. The cascade of different proteins arriving at these structures is signified by different shading of MC. Relative timing of stages and appearance of antigens in the MC is approximate. Full size image It was proposed that parasite membrane proteins are exported to Maurer's clefts by insertion into nascent clefts at the PVM, linking cleft biogenesis and export [2] , [17] , [18] , [22] . Our data indicate that the total number of Maurer's clefts per infected cell is formed very early after invasion and remains constant until shortly before egress. Thus, the clefts are generated before most of the proteins to be exported have been synthesized, and accordingly we show that membrane proteins can reach mature clefts. This suggests that the major route of export for membrane proteins is not via cleft formation but via alternative pathways such as vesicles [24] or soluble intermediates as shown for PfEMP1 [25] . However, if vesicles are involved, they were too small or transient to be detected in our time-lapse experiments. Our findings apply for different types of proteins, the major group of exported proteins containing a PEXEL motif [2] represented by RIFIN-A 29 as well as for PEXEL-negative exported proteins such as SBP1 and REX2 (ref. 53 ). Protein export uncoupled from cleft genesis is more versatile: it allows for an appropriately timed and tuned export cascade to deliver proteins to all Maurer's clefts. Our results do not necessarily exclude that Maurer's clefts derive from the PVM (as they could be generated from this structure in the first 2 h after invasion), but the presence of clefts before detection of the first antigen therein prevents visualization of their genesis and it is possible that they are formed in other ways. Our results link actin with the shape changes seen in ring stages. It is likely that jasplakinolide stabilization had an effect on parasite rather than on host cell actin, as most of erythrocyte actin is already filamentous [54] . However, an effect of the state of erythrocyte actin on parasite shape cannot be entirely ruled out. As myosin is absent from erythrocytes, the BDM results support this; however, inhibitors of better specificity are needed to confirm the role of myosin. The dynamic parasite forms visualized here resemble early descriptions of malaria parasites observed in the blood from patients [26] , but differ significantly from the current view influenced by the widely used fixed and stained parasites or living parasites removed from culture. 4D imaging will pave the way for the study of the dynamic biology of this important pathogen, and to analyse genetically altered parasites and the action of drugs. Plasmid constructs To obtain expression of REX2-GFP under the Mal7P1.170 promoter, 1,714 bp of the 5′ upstream region of the mal7p1.170 gene was PCR-amplified using primers 5′-CATC GCGGCCGC GTAGAACGTTTGGAATATATTCATAG-3′ (restriction sites in primers are underlined) and 5′-CTTGGTAAAAT GGTACC AATTTAATAAAAT-3′ and cloned Not I/ Kpn I into pARL-GFP [55] containing REX2 (pARL-REX2-GFP [37] ), resulting in pARL-REX2-GFP mal7p1.170 . Dendra2 (ref. 46 ) was PCR-amplified from plasmid pDendra2C (a kind gift from Professor Perez, CNRS, Paris) with the primers 5′-AATC CCTAGG ATGAACACCCCGGGAATTAACC-3′ and 5′-TGAC CTCGAG TTACCACACCTGGCTGGGCAGGG-3′, and used to exchange GFP in Avr II/ Xho I-digested pARL-REX2-GFP. To direct GFP to the PV, we cloned the signal peptide of EXP1 into pARL-GFP using primers 5′-CAGC GGTACC ATGAAAATCTTATCAGTATTTTTTCTTGCTC-3′ and 5′-CAGC CCTAGG GCTGCTAACACCACTTCCAGTTCC-3′ to obtain the same fusion protein as previously published [44] . To export GFP into the host cell, we used the amino-terminal part of REX3 (ref. 22 ) that is sufficient to mediate export [43] using primer REX3fwK [37] and reverse primer 5′-CAGC CCTAGG TTTTTTTAAATCCTGTTCTTCTACAAC-3′. Parasite culture and transfection P. falciparum parasites were cultured at a haematocrit of 5% in human 0 + erythrocytes according to standard procedures [56] using RPMI 1640 medium containing 0.5% albumax. Parasites were transfected with 100 μg of purified plasmid DNA using electroporation [57] . Transfectants were obtained after 3–5 weeks' selection with 10 nM WR99210. Synchronization of parasites To obtain highly synchronous parasites that invaded over a defined time window, two protocols were used with comparable results: schizont-stage parasites (3D7 or REX2-GFP crt -expressing parasites) were purified using Percoll [58] , added to fresh erythrocytes in culture medium and then allowed to invade for a defined time window of 1.5–3 h under normal culture conditions. In the first method, Percoll was then used twice to remove the remaining schizonts from the culture to prevent new invasion. In the second method, non-ring-stage parasites were eliminated using sorbitol. Parasites were then washed in media, placed back into culture and samples were removed after regular intervals. Maurer's clefts were counted in at least 30 cells per time point. Tail blood of mice infected with P. berghei was obtained from Rebecca Stanway, BNI, Hamburg. Experiments on mice were carried out in compliance with regulations created and approved by the Ethical Committee of Hamburg state authorities (Nr. FI 28/06). Bodipy-TR-C 5 -ceramide staining Bodipy-TR-C 5 -ceramide (Invitrogen) was prepared according to the manufacturer's protocol to obtain a 5 μM stock solution in PBS and filter-sterilized. For live cell imaging, cells from the parasite culture were removed, washed once in PBS and resuspended in an equal volume of 5 μM Bodipy-TR-C 5 -ceramide solution and incubated for 5 min at 37 °C. Cells were then immediately processed for time-lapse viewing as described under microscopy. For 3D reconstructions of parasites removed from culture, Bodipy-TR-C 5 -ceramide-stained parasites were washed once in RPMI and immediately viewed on a glass slide covered with a coverslip. P. berghei parasites were similarly treated, except that tail blood was washed in RPMI before staining with Bodipy-TR-C 5 -ceramide. Tetanolysin (List Biological Laboratories) lysis was carried out as described [59] . Inhibitor treatments of ring stages Parasites were grown for 1 h in the presence of the indicated concentrations of jasplakinolide (Calbiochem), cytochalasin D (Calbiochem), BDM (Sigma), taxol (Sigma) or colchicine (Sigma) and then immediately viewed blinded by two researchers who counted round and amoeboid parasites. At least 100 cells were counted per condition by each researcher. Identical concentrations of solvent (DMSO or PBS) were used as controls. Immunofluorescence assay Immunofluorescence assays (IFAs) were carried out using infected erythrocytes air-dried on 10-well slides, followed by fixation for 30 min in 100% acetone at room temperature [60] . The wells were rehydrated by three washes in 1× PBS, and the primary antibody was added in blocking solution (3% BSA in PBS) for 1 h. After five washes with PBS, secondary antibody was added in blocking solution for 1 h, followed by five washing steps using PBS. Slides were mounted using Fluorescence Mounting Medium (Dako). Primary antibody dilutions were as follows: mouse monoclonal anti-GFP (Roche): 1/1,000; rabbit anti-REX1: 1/2,500; rabbit anti-SBP1C (a kind gift from Prof Brian Cooke, Monash University, Melbourne, Australia): 1/750; anti-RIFIN A 29 (a kind gift from Drs Michaela Petter and Anna Bachmann; BNI, Hamburg): 1/100. Goat Alexa-Fluor 594 anti-rabbit and Alexa-Fluor 488 anti-mouse (Molecular Probes) were used as secondary antibodies and diluted 1/2,000. Secondary antibody incubations contained 1 μg per ml DAPI (Roche). Microscopy IFAs were analysed using a Zeiss Axioscope M1 microscope (Zeiss) equipped with a 100×/1,4 oil immersion lens and pictures were collected with a Hamamatsu Orca C4742-95 camera (Hamamatsu) and Zeiss Axiovision software (Zeiss). Images were processed in Corel Photo-Paint X3. For time-lapse studies, cells from the parasite culture were arrested on either the glass bottom of a sterile, uncoated, hydrophobic, high, 35 mm μ-Dish (Ibidi) or on a coverslip attached (with fish tank silicone) to a 1 cm 2 hole in the bottom of a 100 ml culture bottle using culture-grade 0.5 mg per ml concanavalin A (Sigma) dissolved in dH 2 O as described [60] . Concanavalin A was added to the glass surface for 10 min, washed off using PBS, and the culture, which was resuspended in PBS, was added and allowed to settle for 5 min. Thereafter, non-bound cells were washed off using PBS, and prewarmed phenol red-free culture medium was added to the dish. Cells were viewed at 37 °C using an Olympus FV1000 confocal microscope equipped with an Olympus Cellcubator (Olympus). Using the multiarea time-lapse function of the Fluoview software and a motorized stage, multiple areas (10–30) of the culture were observed in each experiment. Focus was maintained using the Olympus ZDC autofocus system (Olympus). A 100×/1.4 oil immersion lens and Fluoview software v1.7b was used. Cells were viewed using either 488 nm (GFP and DIC) or 559 nm (Bodipy-TR-C 5 -ceramide and DIC) laser lines. For long-term observations, image collection parameters were usually 4 μs dwell time, 512×512 d.p.i., 16–32 z -stacks (0.2–0.4 μm step size), a zoom level of 1–7 and laser levels of 0.1–3% for 488 nm and 1–5% for 559 nm. Green to red conversion in REX2-Dendra2-expressing cells was achieved using 2,000 μs dwell time of the 405 nm laser with 0.03% intensity restricted to the area containing Maurer's cleft of interest. After conversion, cells were observed as described above. 2D analysis of rapid Maurer's cleft movement in ring stages was carried out using parasites prepared as described for time-lapse imaging but viewed using an QuantEM:512SC EMCCD camera (Spectra Services) mounted onto a Zeiss Observer.Z1 inverted microscope (Zeiss) and imaged using the Zeiss Axiovision software version 4.6 (Zeiss). Data analysis All time-lapse experiments were analysed and processed in Imaris 6.2.0. Cropping of Movies and addition of time stamps were carried out in ImageJ ( http://rsb.info.nih.gov/ij/ ). Single images were processed in Corel Photo-Paint X3. Gauss filters were used with the filter width suggested by Imaris or with a maximum width of 1 pixel in Corel Photo-Paint. How to cite this article: Grüring, C. et al . Development and host cell modifications of Plasmodium falciparum blood stages in four dimensions. Nat. Commun. 2:165 doi: 10.1038/ncomms1169 (2011).